Fine tuning of sub-millisecond conformational dynamics controls metabotropic glutamate receptors agonist efficacy Efficient cell-to-cell communication relies on the accurate signalling of cell surface receptors. Understanding the molecular bases of their activation requires the characterization of the dynamic equilibrium between active and resting states. Here, we monitor, using single-molecule Förster resonance energy transfer, the kinetics of the reorientation of the extracellular ligand-binding domain of the metabotropic glutamate receptor (mGluR), a class C G-protein-coupled receptor. We demonstrate that most receptors oscillate between a resting- and an active-conformation on a sub-millisecond timescale. Interestingly, we demonstrate that differences in agonist efficacies stem from differing abilities to shift the conformational equilibrium towards the fully active state, rather than from the stabilization of alternative static conformations, which further highlights the dynamic nature of mGluRs and revises our understanding of receptor activation and allosteric modulation. Many cell-surface receptors are multimeric multidomain proteins and a better understanding of the underlying molecular mechanisms by which conformational changes regulate their activity is crucial for the development of new innovative drugs. For decades, two models accounting for receptor activation have been widely debated, postulating that either (i) a receptor exists in an equilibrium of a few discrete states, independently of ligand structure and occupancy, and that these states might be differentially stabilized by ligands (conformational selection model), or that (ii) a conformational transition between static states only occurs after a ligand-induced change in shape of the protein (induced fit model) [1] . A validation of one of these models would have important consequences on our understanding of the molecular bases of ligand efficacy. Indeed, partial agonists do not trigger maximized receptor responses, not even at saturating concentrations [2] , a phenomenon that may be explained by either the existence of specific intermediate active conformations, as observed for example for the α-amino-3-hydroxy-5-methyl-4-isoxazole propionic acid (AMPA) receptor [3] , [4] , or by a less efficient shift of the resting-to-active equilibrium with respect to full agonists, as suggested for some N -methyl- D -aspartate (NMDA) receptor partial agonists [5] or nuclear receptors [6] . X-ray crystallography, nuclear magnetic resonance and other structural approaches have been useful to elucidate molecular structures of receptors in various states, but these techniques do not provide sufficient dynamic information on possible transitions between different states to distinguish clearly between these models. Fortunately, spectroscopic techniques performed at the single-molecule level offer the possibility to shed new light on these debates, by directly monitoring conformational changes on individual receptors in real time [7] , [8] . In this study, we quantified, using single-molecule Förster resonance energy transfer (smFRET), the effect of ligands with various efficacies on the resting-to-active transition of metabotropic glutamate receptors (mGluRs). mGluRs are multidomain G-protein-coupled receptors (GPCRs; Fig. 1a ) whose activation mechanism depends on major conformational changes, modulated by the binding of ligands. They are obligate dimers, activated by glutamate [9] , the major excitatory neurotransmitter in the central nervous system, and they are essential to the regulation of synaptic activity [10] , representing, therefore, promising targets in drug development [11] . The eight mGluR subtypes belong to the class C GPCR family, which also includes the receptors for GABA, calcium and for the flavours sweet and umami [12] , [13] . These receptors share a large extracellular ligand-binding domain (ECD), and a heptahelical transmembrane domain (7TM) responsible for G-protein activation ( Fig. 1a ) [11] , [14] , [15] , [16] . Initial structural studies of the isolated ECD dimer revealed that agonist binding in the orthosteric-binding site stabilizes an active (A) state, where the two ECDs are reoriented by 70°, compared with the resting (R) state obtained in the presence of an antagonist ( Fig. 1b ) [17] , [18] , [19] . Yet, other crystal structures have, surprisingly, revealed that the ECD dimer can also adopt either a resting orientation with a bound agonist [16] , or an active orientation in the presence of antagonists, which raises a number of questions regarding the real activation mechanism of these receptors and the mechanism of partial agonism ( Fig. 1c ). 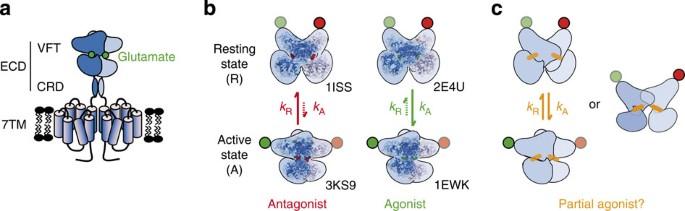Figure 1: Full-length mGluR and the ECD domain in the resting, the active and the putative partially active state. (a) Cartoon representation of the full-length dimeric mGluR. Each subunit is composed of an extracellular bilobate Venus flytrap domain (VFT), forming an interlobe cleft shown to be the orthosteric binding site for ligands, and linked via a cysteine rich domain (CRD) to the transmembrane domain (7TM), responsible for transducing signals to the intracellular C-terminal domain. (b) Overlay of cartoon and molecular envelope representations of the ECD domain of mGluR, observed in the resting (R, top) and in the active (A, bottom) state. ECD domains of various mGluR have been crystallized in the resting state in the presence of antagonist (α-methyl-4-carboxyphenylglycine, PDB:1ISS), or in the active state in the presence of glutamate (PDB : 1EWK). Surprisingly, mGlu1R has also been crystallized in the active state in the presence of the antagonist LY341495 (PDB: 3KS9), and mGlu3R has been observed in the resting state despite the presence of glutamate (PDB: 2E4U). Conformational transitions between these states result in distance variations between the fluorescent labels (SNAP-tags at the N-terminus, green and red dots)21. We definekAandkRas the transition rate constants between these two states. (c) Schematic representation of the potential effect of a partial agonist that could either stabilize less efficiently the active state with respect to the full agonist (left), or alternatively populate an intermediate conformation of the ECD dimer (right). Figure 1: Full-length mGluR and the ECD domain in the resting, the active and the putative partially active state. ( a ) Cartoon representation of the full-length dimeric mGluR. Each subunit is composed of an extracellular bilobate Venus flytrap domain (VFT), forming an interlobe cleft shown to be the orthosteric binding site for ligands, and linked via a cysteine rich domain (CRD) to the transmembrane domain (7TM), responsible for transducing signals to the intracellular C-terminal domain. ( b ) Overlay of cartoon and molecular envelope representations of the ECD domain of mGluR, observed in the resting (R, top) and in the active (A, bottom) state. ECD domains of various mGluR have been crystallized in the resting state in the presence of antagonist (α-methyl-4-carboxyphenylglycine, PDB:1ISS), or in the active state in the presence of glutamate (PDB : 1EWK). Surprisingly, mGlu1R has also been crystallized in the active state in the presence of the antagonist LY341495 (PDB: 3KS9), and mGlu3R has been observed in the resting state despite the presence of glutamate (PDB: 2E4U). Conformational transitions between these states result in distance variations between the fluorescent labels (SNAP-tags at the N-terminus, green and red dots) [21] . We define k A and k R as the transition rate constants between these two states. ( c ) Schematic representation of the potential effect of a partial agonist that could either stabilize less efficiently the active state with respect to the full agonist (left), or alternatively populate an intermediate conformation of the ECD dimer (right). Full size image By labelling the N-terminus of each subunit with FRET compatible fluorophores attached to a SNAP-Tag [20] , the R↔A conformational change has been validated for the full-length mGluRs at the cell surface by a time-resolved luminescence resonance energy transfer (LRET or trFRET) assay [21] . A decrease in the average LRET efficiency was observed in the presence of agonists, in agreement with a reorientation of the ECDs ( Fig. 1b ). High-affinity competitive antagonists reversed this effect, whereas partial agonists lead to a partial decrease in LRET efficacy [21] . Altogether, these investigations established that the ECD dimer can adopt two main conformations, but failed to show why resting and active crystal structures have been observed with bound agonists and antagonists, respectively, as well as the underlying molecular mechanisms leading to partial agonism. In the present study, we address the molecular bases of class C GPCR activation and ligand efficacy by monitoring, at the single-molecule level, the structural dynamics of the dimeric ECD of several mGluR subtypes. Using various advanced procedures to analyse smFRET data, we show that a majority of receptor ECD dimers, whether in their free forms or bound with ligands, oscillate on a hundred microsecond timescale between two main conformations, attributed to the resting and the active state of the receptor. We show that the efficacy of the ligands does not result from a stabilization of specific conformations, but rather from the modulation of the equilibrium constant between the R and the A state. In addition, a small fraction of ECD dimers appear locked in the R or the A state for periods exceeding several milliseconds. This mechanism seems to be conserved for all receptors subtypes, and inspires, therefore, for a new mGluR activation model. Similar activation mechanisms for ECD and full-length mGluRs Before any single-molecule analysis of isolated ECDs, we first verified that the conformational changes associated with the activation of isolated soluble ECD dimers were similar to those observed upon activation of the full-length receptor, using a LRET-based assay [21] . This assay monitors the conformational changes of the dimeric ECD by reporting the distance between the two SNAP-tags labelled with fluorescent substrates (Lumi4-Tb [22] and Green) compatible with LRET measurement [21] . We observed similar LRET changes by agonist stimulation of the full-length mGlu2R ( Fig. 2a ), of mGlu2R-ECD dimers attached to the plasma membrane via a glycosyl phosphatidylinositol (GPI) anchor (mGlu2R-GPI 499 , Fig. 2b ), as for soluble mGlu2R-ECD dimers obtained after cleavage of the GPI anchor with the phosphatidylinositol-specific phospholipase C ( Fig. 2c ), as well as identical K D values. Although glutamate triggered a significant decrease in LRET, the mGlu2R partial agonist DCG-IV only resulted in an intermediate LRET decrease ( Fig. 2 ). Interestingly, all three constructs appear to adopt several conformations even in the absence of ligand. Indeed, the global fit of the delayed emission decays of the acceptor (whose emission is due only to energy transfer received from the long-lived donor [23] , [24] ) requires a triple exponential function. Decay times were 810 and 87 μs, plus a very short component (4 μs) that was neglected because it represented a weak and constant amplitude (<5%), arising from a detector ringing phenomenon [25] . The fraction of the short (87 μs) component (representing species with a high LRET efficiency, that is, in the resting state) decreases similarly for all constructs upon addition of glutamate and, to a lesser extent, in the presence of DCG-IV ( Fig. 2 , right axes, red). These data indicate that the receptor, whether in its full length or ECD form, is most certainly present in several conformations, with a relative abundance governed by the ligand efficacy and concentration. The data also validate the use of soluble ECD dimers obtained after cleavage of the GPI anchor as an excellent model to investigate the conformational dynamics of mGluRs on a single-molecule level. 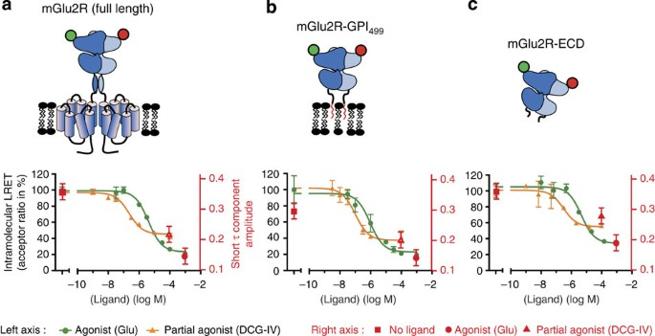Figure 2: Ensemble LRET changes observed within the ECD dimer. The LRET signal, normalized to the maximum signal is represented on the left axis as the ratio of the acceptor-sensitized emissions (see Methods), for SNAP full-length mGlu2R-expressing cells (a), mGlu2R-GPI499-expressing cells (b) or soluble mGlu2R-ECD after GPI cleavage (c). Receptors were labelled with the Lumi4-Tb donor and the Green fluorescent acceptor. The right axis represents the fraction of the short lifetime component obtained by fitting of the acceptor decay that represents the fraction of species with a high LRET efficiency. Binding of the full agonist glutamate leads to a decrease in LRET (•), and the fraction of the short lifetime component (red), as expected for a transition from the resting to the active state (Fig. 1b). Binding of the partial agonist DCG-IV also decreases the LRET (▴) and the fraction of the short lifetime component (red) but to a lower extent, indicating a partial shift of the equilibrium towards the active state, or possibly a stabilization of a partially active intermediate state (see text andFig. 1c). Binding constants are comparable for the cleaved ECD and the full-length receptor (respectively, 4.6 and 4.1 μM for glutamate and 0.31 and 0.23 μM for DCG-IV). Figure 2: Ensemble LRET changes observed within the ECD dimer. The LRET signal, normalized to the maximum signal is represented on the left axis as the ratio of the acceptor-sensitized emissions (see Methods), for SNAP full-length mGlu2R-expressing cells ( a ), mGlu2R-GPI499-expressing cells ( b ) or soluble mGlu2R-ECD after GPI cleavage ( c ). Receptors were labelled with the Lumi4-Tb donor and the Green fluorescent acceptor. The right axis represents the fraction of the short lifetime component obtained by fitting of the acceptor decay that represents the fraction of species with a high LRET efficiency. Binding of the full agonist glutamate leads to a decrease in LRET (•), and the fraction of the short lifetime component (red), as expected for a transition from the resting to the active state ( Fig. 1b ). Binding of the partial agonist DCG-IV also decreases the LRET ( ▴ ) and the fraction of the short lifetime component (red) but to a lower extent, indicating a partial shift of the equilibrium towards the active state, or possibly a stabilization of a partially active intermediate state (see text and Fig. 1c ). Binding constants are comparable for the cleaved ECD and the full-length receptor (respectively, 4.6 and 4.1 μM for glutamate and 0.31 and 0.23 μM for DCG-IV). Full size image smFRET reveals a heterogeneous ensemble of mGlu2R ECD dimers We thus characterized single mGlu2R-ECD dimers freely diffusing in solution, labelled with SNAP substrates carrying the organic fluorophores Cy3B (donor) and d2 (acceptor). We used smFRET with pulsed interleaved excitation (PIE) [26] , [27] and multiparameter fluorescence detection (MFD; Fig. 3a ) [28] , [29] , a technique that provides for each single molecule: its apparent FRET efficiency ( E PR ) calculated from the spectral information, its anisotropy ( r ) determined from the polarization of the photons and the average fluorescence lifetime of the donor dye in the presence of the acceptor ( τ D(A) ). Thanks to the PIE experimental configuration, the average excited lifetime of the acceptor dye ( τ A ) is verified, as well, and only donor–acceptor (D-A) containing complexes are selected based on the stoichiometry factor S PR ( Fig. 3b ) [26] , [30] . 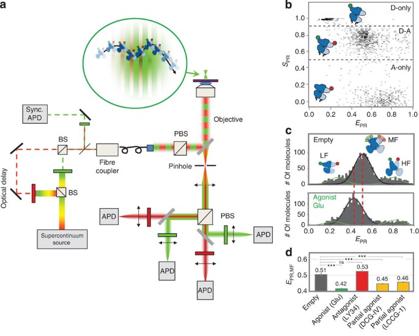Figure 3: PIE-MFD analysis of single diffusing mGlu2R ECD dimers. (a) Schematic illustration of the experimental setup (as described in ref.29). In brief, the output of a pulsed supercontinuum laser is divided into a prompt and a 8-m-long delayed line. Before entering the microscope, the beams are recombined and the pulses are interleaved, generating a multi-colour alternated excitation scheme. For data acquisition, our confocal microscope is equipped with a 4-channel Single Photon Avalanche Diodes detection (APD) and a Single Photon Counting Module (SPCM); (BS, beamsplitter; PBS, polarizing BS). (b) 2D (EPR-SPR) histogram of detected single mGlu2R-ECD dimers in the absence of ligands. D-only and A-only labelled molecules appear with aSPRvalue of ~1 and ~0, respectively, whereas the D-A complexes display an intermediate value (SPR~0.8). Only these D-A complexes are selected for further analysis. (c) TheEPRvalue distribution for the D-A mGlu2R-ECD complexes shows a main population centred aroundEPR=0.51 in the absence of glutamate and two minor populations aroundEPR=0.25 andEPR=0.85 (top). In the presence of glutamate (bottom), theEPRvalue of the main population is shifted towards a lower value (EPR=0.42; see text). (d) Histogram of the mean apparentEPRvalues measured for the dynamic MF population, as a function of the pharmacological nature of the ligand. TheEPRvalue decreased for the agonist, marginally increased for the antagonist, and partially decreased for the partial agonists. Scale bars, s.e.m.,N=10. Figure 3: PIE-MFD analysis of single diffusing mGlu2R ECD dimers. ( a ) Schematic illustration of the experimental setup (as described in ref. 29 ). In brief, the output of a pulsed supercontinuum laser is divided into a prompt and a 8-m-long delayed line. Before entering the microscope, the beams are recombined and the pulses are interleaved, generating a multi-colour alternated excitation scheme. For data acquisition, our confocal microscope is equipped with a 4-channel Single Photon Avalanche Diodes detection (APD) and a Single Photon Counting Module (SPCM); (BS, beamsplitter; PBS, polarizing BS). (b) 2D ( E PR -S PR ) histogram of detected single mGlu2R-ECD dimers in the absence of ligands. D-only and A-only labelled molecules appear with a S PR value of ~1 and ~0, respectively, whereas the D-A complexes display an intermediate value ( S PR ~0.8). Only these D-A complexes are selected for further analysis. (c) The E PR value distribution for the D-A mGlu2R-ECD complexes shows a main population centred around E PR =0.51 in the absence of glutamate and two minor populations around E PR =0.25 and E PR =0.85 (top). In the presence of glutamate (bottom), the E PR value of the main population is shifted towards a lower value ( E PR =0.42; see text). (d) Histogram of the mean apparent E PR values measured for the dynamic MF population, as a function of the pharmacological nature of the ligand. The E PR value decreased for the agonist, marginally increased for the antagonist, and partially decreased for the partial agonists. Scale bars, s.e.m., N =10. Full size image The E PR values observed for (D-A) mGlu2R-ECD show a wide, multimodal distribution ( Fig. 3c ), indicating the co-existence of several conformational states, as inferred from the LRET data. In the absence of ligands, a main population is centred on E PR =0.51 (hereafter designated as the medium FRET population, MF), and two less well-defined minor populations appear around E PR =0.25 and E PR =0.85 (low FRET (LF) and high FRET (HF) populations, respectively). The observation of these minor LF and HF populations does not arise from measurement noise as, for instance, they do not appear on the E PR histogram obtained under similar conditions using a rigid, doubly labelled double-stranded DNA construct ( Supplementary Fig. 1 ). Moreover, the excited state lifetimes of the donor and the acceptor for these three populations match those expected theoretically for doubly labelled complexes engaged in energy transfer ( Supplementary Fig. 2 ). In the presence of glutamate, the E PR value of the MF population decreases significantly ( E PR =0.42, Fig. 3c,d ) as expected for a transition towards the A state of the receptor, whereas the competitive antagonist LY341495 (referred to as LY34 from here onward) reversed this effect ( E PR =0.53, Fig. 3d ). Of note, the E PR values for the LF and the HF states do not appear significantly influenced by the presence of ligands, suggesting that these states remain identical on a macroscopic level. The R↔A transition occurs on a sub-millisecond timescale In order to better define the conformational states from which these three apparent E PR populations originate, we determined the excited-state lifetime of the donor dye for each state. The decays representing the HF, LF and donor-only populations can be described by a single exponential function ( τ D(A), HF =0.5 ns, Fig. 4a ; τ D(A), LF =2.4 ns, Fig. 4c ; τ D =2.7 ns, Supplementary Fig. 3 ). In contrast, the fit of the decay of the MF population requires a double exponential function. Interestingly, the unconstrained fit recovers excited-state’s lifetimes identical to those found for the HF and LF state ( τ =0.5 ns and τ =2.4 ns, Fig. 4b ). This indicates that the molecules belonging to this apparent MF population are not characterized by a fixed D-A distance (single τ D(A) value), but oscillate between the HF and the LF state, at a timescale faster than their diffusion in the observation volume (approximately <4 ms) [31] . Interestingly, the fraction of the long component ( A LF , representing the fraction of molecules from the MF population in the LF state) increases upon addition of glutamate and, to a lesser extent, in the presence of the partial agonists DCG-IV and LCCG-1 ( Fig. 4d ). This observation, fully consistent with the ensemble LRET measurements ( Fig. 2 , right axes), points to the ability of the ligands to influence the HF↔LF equilibrium of the MF population. 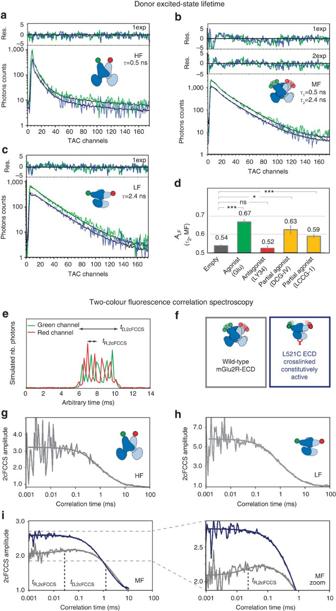Figure 4: Excited-state lifetime and 2c-FCCS analyses. Effect of the L521C mutation. (a–c) The excited-state lifetime of the donor dye is correctly fitted by a single exponential function for the HF (τ=0.5 ns,χ2red=1.23) (a) and the LF (τ=2.4 ns,χ2red=1.19) (c) populations. (b) The mono-exponential fit of the MF population (not shown) does not describe the data in a satisfying manner (τ=1.78 ns,χ2red=1.33, see also weighed residuals above the decays curves,1exp). A better fit is obtained with a bi-exponential decay, which provides the same excited states lifetimes as the mono-exponential fits of the HF and the LF populations (τ1=0.5 ns,AHF=0.22,τ2=2.4 ns,ALF=0.78,χ2red=1.06, see also weighed residuals,2exp). (d)ALFrepresents the fraction of molecules from the MF population in the LF state.ALFincreases upon addition of glutamate and, to a lesser extent, in the presence of the partial agonists DCG-IV and LCCG-1. It is not significantly decreased in the presence of antagonist. Scale bars, s.e.m.,N=5. (e) Principle of the two-colour cross-correlation spectroscopy (2cFCCS) analysis: if a molecule switches between a high FRET and a lower FRET state at a timescale (tR) faster than its diffusion (tD) across the observation volume, the photons detected in the green and red emission channels are anticorrelated.tDandtRwill appear as positive and negative contributions, respectively, on a 2cFCCS curve. (f–i) 2cFCCS analysis. Anticorrelation between photons detected in the green and in the red channels is clearly observed for the MF population of the WT-ECD (h, grey) as expected for a LF↔HF transition, at the 50–100 μs timescale. This anticorrelation disappears for the L521C construct (f–i, blue), indicating a reduction of its conformational dynamics compared with the WT-ECD, and is not present for the static HF (g) or LF (h) populations. Figure 4: Excited-state lifetime and 2c-FCCS analyses. Effect of the L521C mutation. ( a – c ) The excited-state lifetime of the donor dye is correctly fitted by a single exponential function for the HF ( τ =0.5 ns, χ 2 red =1.23) ( a ) and the LF ( τ =2.4 ns, χ 2 red =1.19) ( c ) populations. ( b ) The mono-exponential fit of the MF population (not shown) does not describe the data in a satisfying manner ( τ =1.78 ns, χ 2 red =1.33, see also weighed residuals above the decays curves, 1exp ). A better fit is obtained with a bi-exponential decay, which provides the same excited states lifetimes as the mono-exponential fits of the HF and the LF populations ( τ 1 =0.5 ns, A HF =0.22, τ 2 =2.4 ns, A LF =0.78, χ 2 red =1.06, see also weighed residuals, 2exp ). ( d ) A LF represents the fraction of molecules from the MF population in the LF state. A LF increases upon addition of glutamate and, to a lesser extent, in the presence of the partial agonists DCG-IV and LCCG-1. It is not significantly decreased in the presence of antagonist. Scale bars, s.e.m., N =5. ( e ) Principle of the two-colour cross-correlation spectroscopy (2cFCCS) analysis: if a molecule switches between a high FRET and a lower FRET state at a timescale ( t R ) faster than its diffusion ( t D ) across the observation volume, the photons detected in the green and red emission channels are anticorrelated. t D and t R will appear as positive and negative contributions, respectively, on a 2cFCCS curve. ( f – i ) 2cFCCS analysis. Anticorrelation between photons detected in the green and in the red channels is clearly observed for the MF population of the WT-ECD ( h , grey) as expected for a LF↔HF transition, at the 50–100 μs timescale. This anticorrelation disappears for the L521C construct ( f – i , blue), indicating a reduction of its conformational dynamics compared with the WT-ECD, and is not present for the static HF ( g ) or LF ( h ) populations. Full size image Measuring the excited state lifetime is a straightforward method to estimate the D-A distances for the LF and the HF state. Assuming a R 0 value of 54 Å, we measured R DA,LF,Lif =73±4 Å and R DA,HF,Lif =42±2 Å, respectively. To compare these values with those theoretically expected for the active and the resting state, we simulated the fluorophores positions on a model of a SNAP-ECD dimer based on the crystal structures of mGlu1R. We found very broad distributions, differing significantly between the A and R conformations, in agreement with the LRET and smFRET measurements ( Supplementary Fig. 4 ). The difference in the mean theoretical inter-dye distance calculated between these two conformations (~10 Å) appears smaller than those measured experimentally (31±6 Å), however, this theoretical mean value might be biased for several reasons (see Supplementary Fig. 4 ). Altogether, we propose that a majority of mGluR ECDs, belonging to the MF population, oscillate between two states representing conformations close to the A and R states observed in crystallography. In addition, at the timescale of our measurement (<4 ms), minor populations of the ECD-dimers appear blocked in a static LF-active state (hereafter named A S ) or in a static HF-resting state (named R S ). To confirm this hypothesis, we performed a correlation analysis of the fluctuations of the fluorescent signals over time for the various subpopulations (see experimental details in Supplementary Note ). The two-colour cross-correlation spectroscopy analysis (2cFCCS) is a powerful statistical tool to unveil conformational fluctuations at short timescales [32] , [33] , [34] . For a dynamic system undergoing FRET changes at a faster-than-diffusion timescale, anti-cross-correlation, at short timescales, should theoretically be observed between photons detected in the green and in the red channels (see illustration on Fig. 4e ), although this effect is rarely observed experimentally. A clearly visible anticorrelation effect is observed at short timescales for the MF species ( Fig. 4i ), whereas no anticorrelation is visible for the LF and HF subpopulations ( Fig. 4g,h ). Similar curves were obtained for all investigated ligands (not shown), and were fitted with equation (1): where N is the average number of molecules in the observation volume, t D is their diffusion time, ω 0 and z 0 are the 1/ e 2 radii of the laser focus volume perpendicular to and along the optical axis, respectively, A R,2cFCCS and t R,2cFCCS represent the amplitude and the relaxation time, respectively, of the dynamic transition observed only in the case of the MF population. The exact t R,2cFCCS value could not be determined with high accuracy because of high noise levels in the 2cFCCS data, but it appeared to be in the 20–100 μs range. Our 2cFCCS data underline the dynamic nature of the MF population, which oscillates rapidly between two states. It is tempting to assign these two states to the HF (R) and the LF (A) state, based on the excited states lifetimes measured for the MF population. To verify this hypothesis, we employed filtered FCS (fFCS), a method used to separate the correlation functions of individual components of a mixture with different FRET-states [35] based on their differences in fluorescence lifetime, polarization and spectral properties [36] (see experimental details in Supplementary Note ). Three component fluorescence filters for fFCS were generated using decay patterns from scatter (buffer), and from HF and LF subpopulations, and we calculated the probability for each photon to belong to one of these three states ( P (scatter) , P (LF) , P (HF), see Fig. 5a for illustration). Species cross-correlation functions (SCCFs) between HF and LF components display a positive cross-correlation diffusion term, indicating that a substantial fraction of molecules effectively undergo LF↔HF transitions during their residence in the observation volume. The clearly visible anti-cross-correlation term at short timescales (50–100 μs) represents the relaxation time for the LF↔HF transition ( Fig. 5b ). SCCF curves were globally fitted applying equation 1, where A R,2cFCCS and t R,2cFCCS are replaced with A R,SCCF and t R,SCCF , representing the amplitude and the relaxation time of the LF↔HF transition, respectively. Similar to the 2cFCCS measurements, the order of magnitude of these relaxation times is in the ~100 μs range in the absence or presence of ligands ( Table 1 ). The fraction of molecules undergoing fast A↔R transition ( A R,SCCF ) is not visibly affected by the ligands ( Fig. 5d and Table 1 ). 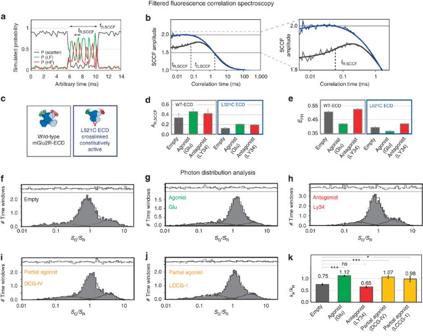Figure 5: Filtered FCS (fFCS) and photon distribution analyses (PDA). Effect of the L521C mutation. (a) Principle of the fFCS analysis: a probability is assigned to each photon to belong to either the scattering signal (P(scatter)), to the low FRET state (P(LF)) or to the high FRET state (P(HF)). If a molecule switches between the LF and the HF state at a timescale (tR) faster than its diffusion across the observation volume (tD), the probabilities of the photons belong to the LF or the HF state are anticorrelated.tDandtRwill appear as positive and negative contributions, respectively, to the Species Cross Correlation Function (SCCF) curve. (b) SCCF curves calculated using full photon streams for the WT-ECD (grey) and the constitutively active L521C (blue) receptor. The anti-cross-correlation term represents the relaxation timetR,SCCFfor the LF↔HF (and thus the A↔R) transition. (c,d) The amplitude of the anticorrelation term is strongly reduced for the L521C mutant (blue), indicating a reduction of its conformational dynamics with respect to the WT-ECD (grey). (e) Histogram of theEPRvalues for the MF species, as a function of the ligand, for the WT-ECD (grey, left) and the L521C mutant (blue, right). For all ligands tested, theEPRvalues for the L521C mutant are equal or lower than the ones observed for the WT-ECD activated by glutamate, in accordance with the constitutively active character of the L521C mutant. (f–j) PDA histograms (expressed as uncorrectedSG/SRratios) of single mGlu2R ECD dimers, in the presence of various ligands. Data were fitted (black lines) with a model that accounts for two static species (HF,SG/SR=0.2 and LFSG/SR=3), and a dynamic species interconverting between these states (MF,SG/SR=0.8–1.2, depending on the ligand). (k) Histogram of the mean apparentkA/kRvalues calculated from the fit of the PDA histograms. Agonist binding leads to a strong increase of thekA/kRratio compared with the empty receptor. Antagonist binding only marginally pushes the equilibrium in the opposite direction. Interestingly, partial agonists push the equilibrium significantly towards the Active state, but with less efficiency than the full agonist glutamate. Figure 5: Filtered FCS (fFCS) and photon distribution analyses (PDA). Effect of the L521C mutation. ( a ) Principle of the fFCS analysis: a probability is assigned to each photon to belong to either the scattering signal (P(scatter)), to the low FRET state (P(LF)) or to the high FRET state (P(HF)). If a molecule switches between the LF and the HF state at a timescale ( t R ) faster than its diffusion across the observation volume ( t D ), the probabilities of the photons belong to the LF or the HF state are anticorrelated. t D and t R will appear as positive and negative contributions, respectively, to the Species Cross Correlation Function (SCCF) curve. ( b ) SCCF curves calculated using full photon streams for the WT-ECD (grey) and the constitutively active L521C (blue) receptor. The anti-cross-correlation term represents the relaxation time t R,SCCF for the LF↔HF (and thus the A↔R) transition. ( c , d ) The amplitude of the anticorrelation term is strongly reduced for the L521C mutant (blue), indicating a reduction of its conformational dynamics with respect to the WT-ECD (grey). ( e ) Histogram of the E PR values for the MF species, as a function of the ligand, for the WT-ECD (grey, left) and the L521C mutant (blue, right). For all ligands tested, the E PR values for the L521C mutant are equal or lower than the ones observed for the WT-ECD activated by glutamate, in accordance with the constitutively active character of the L521C mutant. ( f – j ) PDA histograms (expressed as uncorrected S G /S R ratios) of single mGlu2R ECD dimers, in the presence of various ligands. Data were fitted (black lines) with a model that accounts for two static species (HF, S G /S R =0.2 and LF S G /S R =3), and a dynamic species interconverting between these states (MF, S G /S R =0.8–1.2, depending on the ligand). ( k ) Histogram of the mean apparent k A / k R values calculated from the fit of the PDA histograms. Agonist binding leads to a strong increase of the k A / k R ratio compared with the empty receptor. Antagonist binding only marginally pushes the equilibrium in the opposite direction. Interestingly, partial agonists push the equilibrium significantly towards the Active state, but with less efficiency than the full agonist glutamate. Full size image Table 1 Parameters extracted from the fit of the smFRET data obtained for mGlu2R. Full size table Altogether, our results obtained using two independent correlation methods (fFCS and 2cFCCS) demonstrate that the molecules belonging to the MF population undergo fast (50–100 μs) transitions between the A and the R state. Importantly, we noted that these fast relaxation events observed in the correlation analysis do not arise from fluorophore photophysics (blinking; see Supplementary Fig. 5 ). In addition, we verified that the various FRET distributions and FRET changes do not originate from artefacts because our labelling strategy, as the use of other fluorophore pairs or other labelling approaches provided similar results (see Supplementary Fig. 6 ). A shift towards the A state in a constitutively active mutant We recently demonstrated that a specific crosslinking with an intersubunit disulfide bond (mGlu2R-L521C, Fig. 4f ) leads to a constitutively active receptor dimer [14] . The ECD of this mutant shows an E PR distribution qualitatively similar to the one observed for the wild-type (WT)-ECD activated by glutamate, indicating that the A↔R equilibrium is preferentially shifted towards the active form for the mutant. The apparent E PR value of the MF population is close to that obtained with the WT-ECD construct in the presence of agonist ( E PR =0.39±0.01 versus E PR =0.42±0.01, respectively), whereas the antagonist (LY34) or the agonist glutamate only marginally altered this E PR value ( Fig. 5e , Table 1). Correlation analyses also clearly show a reduction of the amplitude of the LF↔HF transition term for the mutant with respect to the WT-ECD, both in the fFCS analyses ( Fig. 5b , compare blue and grey curves, respectively, and Fig. 5e ), and the 2cFCCS measurements ( Fig. 4i ). Altogether, our data demonstrate a strong reduction of the conformational dynamics of the ECD, and a shift of the A↔R equilibrium towards the active state, in agreement with the constitutive activity of this mutant mGluR. Ligand binding influences the R↔A transition rates In order to estimate the rate constants of the fast HF ↔ LF transition, we used a photon distribution analysis (PDA) approach, a method that quantitatively and precisely describes the FRET signal distribution [37] , [38] . PDA has already been successfully implemented to discriminate between multiple species coexisting in solution and to highlight dynamic behaviour of single molecules [38] , [39] , [40] . Figure 5f–k represents the signal intensity ratio distribution from the green and red detection channels ( S G and S R , respectively) for the mGlu2R-ECD dimers. The three populations appear at low, medium and high S G / S R ratios (for HF, MF and LF, respectively). By applying a simple PDA two-state dynamic model, taking into account two minor populations (HF and LF), presumably static at the measurement timescale (~4 ms), and a major MF population composed of molecules undergoing sub-millisecond interconversions between these two boundary states, the experimental distribution was accurately described ( Fig. 5f–j ). The choice of this dynamic PDA model ( Supplementary Fig. 7 ) is fully supported both by the correlation and excited state lifetime analyses ( Figs 4 and 5 ). In addition to the apparent FRET efficiency ( E PR ) for these states, the PDA model provides the fraction of molecules for the LF, HF and apparent MF populations, and k A and k R , the rates constants of the transitions towards the active and resting state, respectively. The D-A distances measured by PDA for the LF and HF populations match those measured by analysing the excited-state lifetime of the donor. For the LF species, the agreement is perfect ( R DA,LF,PDA =76±13 Å versus R DA,LF,Lif =73±4 Å), whereas for the HF species, a slight difference is observed ( R DA,HF,PDA =31±6 Å versus R DA,HF,Lif =42±2 Å), possibly due to an overestimation of the donor lifetime at very high FRET efficiencies as a result of the small number of emitted photons. The shift in equilibrium between R and A states triggered by the ligands for the MF population correlates with drug efficacy, as quantified by calculating the k A / k R ratio ( Fig. 5k ). The observed effects of the ligands are in full agreement with what was previously determined from the apparent E PR,MF value ( Fig. 3d ), and from calculating the fraction of molecules transiently in the HF state from the fit of the excited state decay of the MF population ( A HF , Fig. 4d; see also Table 1 ). For example, a saturating concentration of glutamate shifts the R↔A equilibrium towards the A state with respect to the empty receptor, as shown by an increase of the k A / k R ratio, and a decrease in the E PR,MF and A HF values ( Figs 3d and 4d ), as observed in ensemble LRET analyses ( Fig. 2c and see ref. 21 ). Conversely, binding of the antagonist LY34 did not lead to any significant changes, although a slight increase in the apparent E PR,MF and A HF values and a modest decrease of the k A / k R ratio were detected. Interestingly, it appears that agonists potencies correlate with their ability to push the R↔A equilibrium towards the A state. Indeed, for the partial agonists DCG-IV and LCCG-1, the apparent E PR,MF and A HF values decreased, and the k A / k R ratio increased, as with glutamate, but to a lesser extent ( Figs 3d , 4d and 5k and Table 1). This finding highlights the partial character of these ligands, which seem to less efficiently shift the conformation equilibrium towards the A state, in comparison with the full agonist. This is not consistent with a model where the partial agonist merely stabilizes an alternative conformation, different from the fully active state populated in the presence of a full agonist. An activation mechanism conserved for all mGluR subtypes Based on their sequence conservation and pharmacological properties, the eight mGluRs can be divided into three groups [10] : Group I is represented by mGlu1R and mGlu5R; group II comprises mGlu2R and mGlu3R; and all the other members belong to group III. mGluRs of the same group show about 70% sequence identity, whereas between groups this percentage decreases to about 45%. We found that the conformational dynamics linked to mGluR ECD dimer activation described here for mGlu2R are conserved for mGlu4R and mGlu5R, representing other receptors subgroups. E PR distributions obtained with these receptors matched those obtained with mGlu2R, although the exact E PR values differed, because of different structures of the complexes. Glutamate binding resulted in a decrease in the apparent E PR value of the MF population ( Fig. 6a ) and an increase of the k A / k R ratio ( Fig. 6b ), which are reversed by a competitive antagonist. In addition, binding of the mGlu4R partial agonist γ-carboxy- L -glutamate (Gla) leads to a slight decrease of the apparent E PR value, whereas the increase of the k A / k R ratio is too weak to be considered significant, in full agreement with the weak activity of this ligand [41] . Finally, fFCS analyses also point to a fast (<1 ms) switching for both types of receptor dimers between the A and the R states ( Fig. 6c ), as observed for mGlu2R. 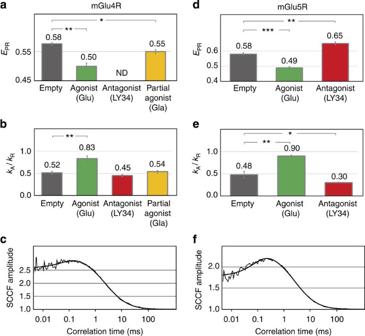Figure 6: MFD, PDA and fFCS analyses of single diffusing mGlu4R (left) and mGlu5R (right) ECD dimers. (a,d) Histogram of the mean apparentEPRvalues measured for the dynamic MF species, as a function of the nature of the ligand, mGlu4R (a) and mGlu5R (d). For both receptor subtypes, theEPRvalues decrease upon agonist or partial agonist binding, and increase upon antagonist binding, although the exactEPRvalue for mGlu4R in the presence of antagonist was too high to be determined. (b,e) Accordingly,kA/kRvalues increase upon agonist binding, and decrease upon antagonist binding, reflecting the shift of the A↔R equilibrium induced by the ligands. (c,f) SCCF analyses show a negative cross-correlation as sub-milliseconds timescales term representing the LF↔HF (and thus the A↔R) transition. The order of magnitude of these relaxation times is similar to those found for mGlu2R. Figure 6: MFD, PDA and fFCS analyses of single diffusing mGlu4R (left) and mGlu5R (right) ECD dimers. ( a , d ) Histogram of the mean apparent E PR values measured for the dynamic MF species, as a function of the nature of the ligand, mGlu4R ( a ) and mGlu5R ( d ). For both receptor subtypes, the E PR values decrease upon agonist or partial agonist binding, and increase upon antagonist binding, although the exact E PR value for mGlu4R in the presence of antagonist was too high to be determined. ( b , e ) Accordingly, k A / k R values increase upon agonist binding, and decrease upon antagonist binding, reflecting the shift of the A↔R equilibrium induced by the ligands. ( c , f ) SCCF analyses show a negative cross-correlation as sub-milliseconds timescales term representing the LF↔HF (and thus the A↔R) transition. The order of magnitude of these relaxation times is similar to those found for mGlu2R. Full size image Over the years, several models have emerged to account for the molecular mechanisms that govern receptor activation. In particular, two conflicting theories postulating either a conformational selection or an induced fit mechanism have drawn much attention and been widely debated. In line with this debate, the molecular basis of the partial agonism observed for certain ligands remain obscure. Here, using the ligand binding domain of mGluRs, we presented a smFRET study that reveals surprisingly fast structural dynamics, on a sub-millisecond timescale, corresponding to transitions between an activated and a resting state. These observations motivated us to put forward a new model for mGluR activation ( Fig. 7 ), in which ligands finely tune the conformational dynamics of the receptor rather than stabilizing specific conformations. 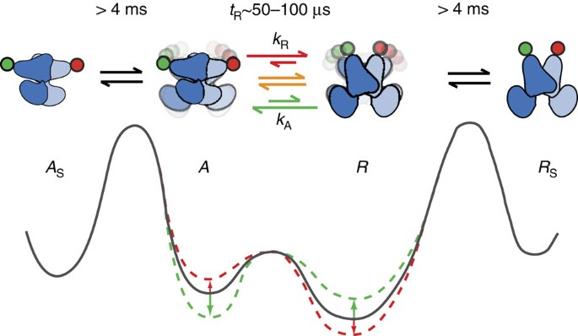Figure 7: Proposed model for mGluR activation. The mGluR ECD dimer exists in a preformed equilibrium of conformational states, interconverting at a 50–100 μs timescale and the exclusive role of ligands is to modulate the transition rates between these states (green, effect of an agonist; red : effect of an antagonist). A fraction of the ECD dimers appear static in aRSor in aASstate. A conformational transition between these static states, and the dynamic states would only occur at a timescale longer than our observation time, that is, ~4 ms. Figure 7: Proposed model for mGluR activation. The mGluR ECD dimer exists in a preformed equilibrium of conformational states, interconverting at a 50–100 μs timescale and the exclusive role of ligands is to modulate the transition rates between these states (green, effect of an agonist; red : effect of an antagonist). A fraction of the ECD dimers appear static in a R S or in a A S state. A conformational transition between these static states, and the dynamic states would only occur at a timescale longer than our observation time, that is, ~4 ms. Full size image Our data refute a simple static activation model, where the binding of a ligand triggers a conformational change of the receptor towards a static state. Instead, we show that the mGluR ECD dimer is in a constant and fast dynamic exchange between at least two states, whether unbound or bound by an agonist or an antagonist. The LF and the HF state correspond to conformations where the receptor is preferentially either active or resting, respectively. The vast majority of molecules display an apparent intermediate (MF) E PR value that is influenced by the pharmacological nature of the ligand. This population does not correspond to a static state, as demonstrated by measuring the excited state lifetime of the donor dyes ( Fig. 4a–c ), by 2cFCCS analyses ( Fig. 4d–i ), by fFCS measurements ( Fig. 5a,b ) and by fitting the E PR distribution using a dynamic PDA model considering two interconverting states ( Fig. 5f–j ). In addition, a minority of molecules appear static at high or low E PR values implying that these molecules reside in a stabilized resting ( R S ) or active ( A S ) state for a period of time exceeding the residence time in the observation volume, that is, >4 ms ( Fig. 7 ). It cannot be excluded that these molecules are in reality in slow exchange with the population of dimers engaged in the fast A↔R exchange, even though this could not be examined in our study. Determining whether the exploration of the A S state is required for the activation of the receptor in its native environment and proper signal transduction will be the subject of a future study using full-length receptors reconstituted in lipid nanodiscs [9] , an approach successfully used in FCS studies of other membrane proteins [42] , [43] . Our data explain how mGluR ECDs could be crystallized in an ‘active’ conformation despite antagonist binding (PDB 3KS9, Structural Genomics Consortium,) and in a ‘resting’ conformation in the presence of an agonist [16] . In fact, as the R and A state are in rapid exchange and are energetically close even in the presence of ligands ( Fig. 7 ), crystallization of a receptor dimer in any of these two states could easily be envisioned. Given the nature of our experiments, which solely report on the distance between two points located close to the N-termini of the receptor ECD dimer, it is conceivable that the HF and the LF state in reality represent several sub-states, for which the distance between the N-termini in the dimer is similar. Although this hypothesis cannot be formally ruled out, these potential sub-states would not result in significantly different activation efficacies, given the excellent correlation reported between: (i) the estimated relative populations of the HF and LF states (measured from donor excited-state lifetime measurements ( Fig. 4d ) or PDA analysis ( Fig. 5k )); (ii) the distance measurements by ensemble LRET between the N-terminal SNAP-tags on the full-length receptors ( Fig. 2 and ref. 21 ); and (iii) cellular functional assays based on inositol phosphate accumulation and calcium mobilization [21] . The conformational transitions between the R and the A state occur on a ~100-μs timescale ( Fig. 7 ). The ligands influence the transition rates between these states, increasing thus the probability of the receptor to reside in one of them, although these effects appear very subtle (see k A / k R analysis, Fig. 5k ). This type of mechanism, characterized by the exploration of a conformational space, and where the ligand influences the probability of entering a given state has also been observed on the isolated monomeric glutamate binding domain of the GluA2 subunit of the AMPA receptor [44] . Similarly, the full-length β 2 -adrenergic receptor (β 2 AR), a class A GPCR, has been shown to explore a conformational space in the presence of various ligands that bind in the 7TM domain [45] , [46] . The estimated relaxation times spanned the microseconds to seconds range, and the equilibrium was fully shifted towards the active state only in the presence of the G-protein mimic nanobody Nb80 (refs 45 , 46 ). The proposed activation model also highlights the molecular mechanism of partial receptor activation by some ligands. In vivo, DCG-IV has a partial effect on mGlu2R estimated to be roughly 80% of that of glutamate, whereas that of LCCG-1 is slightly lower, about 70% (ref. 21 ). Interestingly, the tendency of LCCG-1 to show a slightly lower effect than DCG-IV was detected throughout our smFRET experiments, highlighting the correlation between the k A / k R ratio of the various agonists determined by PDA and their potency for receptor activation. This effect is also observed for γ-carboxy- L -glutamate (Gla), a weak activator of mGlu4R [41] , whose effect on the k A / k R ratio is correspondingly very limited ( Fig. 6b ). Our model proposes that partial agonists are able to push the R ↔ A equilibrium towards the fully activated state, but to a lesser extent than glutamate. This finding is consistent with disulfide trapping experiment on the related GluA2 subunit of the AMPA receptor, for which a fully closed form of the LBD can be obtained in the presence of partial agonists [47] . It also explain the identical conformations observed by X-ray crystallography for mGlu3R both in the presence of glutamate and DCG-IV [16] , even though the latter has been shown to act as a partial agonist on mGlu3R in LRET experiments [21] . The prominent role of structural dynamics in GPCR function is now generally accepted (reviewed in ref. 48 ), and even though the model we propose here to explain the molecular basis of partial agonism in the case of mGluRs seems sufficient, the mechanisms accounting for the effect of partial ligands for non-class C GPCR is still a matter of debate. Early biophysical experiments, mainly performed on β 2 AR, led to conflicting conclusions. Indeed, some environment-sensitive fluorescent probes reported differently to partial and total agonists, but this variable effect was only detected for a subset of positions of the probes on the receptor [49] , [50] , [51] , [52] . Moreover, in some cases, the signal variation detected in the presence of partial agonists could be explained by an incomplete stabilization of the fully active state, rather than by the existence of an alternative static conformation. Yet, it appears that for some ligands the local conformational changes triggered by their binding to the 7TM domain could account for their partial activity. For example, fluorescence and structural modelling studies have shown that the partial agonist salbutamol promoted an alternative conformation of β 2 AR because of a different binding mode with respect to the cognate catecholamine full agonist [53] . Finally, it also has been proposed that the partial activity of some agonists could stem from their differential ability to promote a stable ternary complex (agonist/β 2 AR/nucleotide-free G α protein) [54] . Our smFRET data are in very good agreement with the ensemble in cellulo LRET data regarding the general activation mechanism of the full-length mGluR ( Fig. 2 ). Interestingly, the existence of several populations has been inferred from these LRET data, as an accurate fit of the acceptor-sensitized emission decay on the full-length construct requires a triexponential function, which clearly favours the existence of several populations in cellulo . We cannot exclude that the presence of the trans-membrane domain in the full-length receptor influences the kinetics of the A↔R equilibrium. However, recent experiments suggest that the dimeric ECD domain is the dominant element when it comes to regulating the conformational changes that occur within the 7TM domain and which lead to G-protein activation. Indeed, the glutamate affinity on the isolated ECDs is very similar to that determined on the full-length receptor [51] , [55] , [56] , [57] . Moreover, we showed that on a an isolated 7TM domain of mGlu2R and on a full-length monomeric mGlu2R construct reconstituted in lipids nanodiscs, positive and negative allosteric modulators acted as full agonists and antagonists, whereas glutamate alone had no effect [9] . The activation of the G-protein by glutamate was recovered upon using of the full-length dimeric receptor, underlying the key role of the ECDs, as a dimer, in the activation process [9] . In summary, we clearly demonstrate that the extracellular domain of the mGluR exists in a preformed equilibrium of conformational states and that the exclusive role of ligands is to modulate the transition rate between states, rather than stabilizing individual conformations at the expense of others. The observation that ligands finely tune conformational dynamics is consistent with other studies carried out on membrane receptors, including ligand-gated ion channels [58] and class A GPCRs [45] , [46] , [59] . Our results, using the extracellular domain of mGluRs as a model system, inspire for a new mechanism describing the activation of cell surface receptors as a stochastic process where the probability of activation is intrinsically linked to the frequency of the conformational changes towards the activated state. Materials Glutamate was purchased from Sigma-Aldrich. LY341495 was acquired from Abcam Biochemicals and DCG-IV ((2S,2′R,3′R)-2-(2′,3′-Dicarboxycyclopropyl) glycine) and LCCG-1 ((2S,1′S,2′S)-2-(Carboxycyclopropyl)glycine), from Tocris Bioscience. Lipofectamine 2000 was bought from Life Technologies. CoA-547 and CoA-647 were purchased from NewEngland BioLabs. SNAP-Lumi4-Tb and SNAP-Green were obtained from Cisbio Bioassays. Benzylguanine-Cy3B and benzylguanine-d2 Benzylguanine-d2 (ref. 60 ) was prepared according to the literature by Cisbio Bioassays. Benzylguanine-cy3B was synthesized by adding aminomethylbenzamide-benzyl guanine (1 μmol) dissolved in anhydrous dimethylsulfoxide (100 μl) to N,N -diisopropylethylamine (1 μl–5.7 μmol) and a solution of Cy3B-NHS (GE Healthcare Life Sciences, 1 μmol) in anhydrous dimethylsulfoxide (270 μl). The mixture was stirred at room temperature for 1 h. Purification was performed by preparative HPLC to give the desired conjugate evaluated by OD (355 nmol, 35%). High Resolution Mass Spectrometry (ESI + ) Calcd for C 52 H 53 N 9 O 7 S [M+H] 2+ : m/z 473.6891, found 473.6888. Transfection, purification and labelling pcDNA3 plasmids encoding the Flag-SNAP-tagged human mGlu2R-499GPI and human mGlu2R-561GPI were provided by Cisbio Bioassays. The single point mutations generating the mGlu2R,L521C-561GPI constructs were generated using the QuikChange mutagenesis protocol (Agilent Technologies). HEK-293 cells were cultured in DMEM (Life Technologies) supplemented with 10% fetal calf serum (Lonza). HEK-293 cells were transfected by the reverse Lipofectamine 2000 protocol in 24-well Petri-dishes (Becton-Dickinson) for 48 h before incubation at 37 °C for 1 h with a solution containing 1 μM Benzyl-Guanine-d2 and 10 nM Benzyl-Guanine-Cy3B, and washed three times with filtered TK buffer, pH 7.4. (Tris-HCl, pH 7.4, 20 mM, NaCl 125 mM, KH 2 PO 4 1.2 mM, MgSO 4 1.2 mM, KCl 4.5 mM, CaCl 2 2 mM). The GPI-anchor was cleaved by adding 0.25 U ml −1 Bacillus cereus Phosphatidylinositol-specific Phospholipase C (Invitrogen, P8804) and incubated for 45 min at 37 °C. The supernatant was desalted using ZebaTM desalt spin columns (Fisher Scientific) and stored at −20 °C supplemented with 50% glycerol and 0.1 mg ml −1 BSA. Occasionally, an anti-flag purification preceded desalting, in which case an ANTI-FLAG M1 Agarose Affinity Gel was used (Sigma-Aldrich) following the provided standard protocol. For LRET measurements, cells were transfected by electroporation or by the reverse Lipofectamine 2000 protocol [21] . Cells were incubated at 37 °C for 1 h with a solution of 300 nM SNAP-fluorophore and were washed three times with tag-Lite buffer [21] . LRET experiments The LRET measurements were performed in Greiner black 96-well plates on a PHERAstar FS microplate reader with the following setup: after excitation with a laser at 337 nm (40 flashes per well), the fluorescence was collected at 520 nm for a 50-μs reading after a 50-μs delay after excitation (window 1) or for a 400-μs reading after a 1,200-μs delay (window 2). The acceptor ratio was determined by dividing the signal measured in window 1 by the signal measured in window 2 and then was plotted on logarithmic scale. The intensity level of window 2 was above noise level by at least a factor of 5 to avoid erroneous divisions. We chose this representation because, in the range of acceptor ratio measured, the log of the ratio is correlated linearly with the distance between Lumi4Tb and Green. The delayed emission decays of the acceptor were fitted using the GLOBALS software (Laboratory for Fluorescence Dynamics, Irvine, CA) using a triple exponential decay function. The value of the excited state lifetimes were linked and fitted globally, whereas the amplitude of the various preexponential factors were allowed to vary freely. Molecular fractions presented in Fig. 2 were calculated from the preexponential factors and the excited state lifetime values as described in Heyduk and Heyduk [24] . Multiparameter fluorescence detection setup and FRET-measurements Single-molecule FRET measurements were performed on our home-built confocal PIE-MFD microscope as described in Olofsson et al. [29] , in 384-well plates (Greiner Bio One) at a concentration of approximately 20–50 pM. All samples were prepared in filtered TK buffer, pH 7.4 and ligands were added at saturating concentrations. 40–60 million photons, corresponding to an acquisition time of roughly 2.5 h, were collected per experiment and further analysed with the Software Package for Multiparameter Fluorescence Spectroscopy, Full Correlation and Multiparameter Fluorescence Imaging developed in C.A.M. Seidel lab ( http://www.mpc.uni-duesseldorf.de/seidel/ ). A single-molecule event was defined as a burst containing at least 40 photons with a maximum allowed interphoton time of 0.3 μs and a Lee-filter of 20. Molecules were selected for further analysis only if the following criteria were fulfilled: 0.6< S for the removal of acceptor-only labelled molecules, 1.5 ns< τ A <2.5 ns for the removal of donor-only labelled molecules and |T GX -T RR |<0.75 ms to eliminate photobleaching events as described in ref. 28 . The ECD dimer was further purified using the Flag-tag inserted in N-terminus of the construct, and single-molecule FRET results on this purified fraction were similar to those obtained on the supernatant, highlighting the excellent specificity of the Snap-tag labelling procedure (data not shown). Thus, for the remaining part of the study, measurements were conducted directly following PI-PLC cleavage without any further purification steps. PDA analysis In order to further resolve and quantify heterogeneities within the measured FRET distributions, PDA was employed ( Fig. 4 ). For this analysis each burst is divided into time windows (t.w.) and then for each t.w., the fluorescence parameters are calculated. PDA is a powerful technique that allows for the determination of the minimum width of a FRET distribution arising from a single interdye distance. This minimum width is determined by the photon shot noise, which arises from the fact that the number of photons detected per single-molecule burst is relatively small (typically a few hundreds of photons). PDA has already been successfully implemented to discriminate between multiple species coexisting in solution and to highlight dynamic behaviour of single molecules just by applying the model of static states to histograms of different t.w. In fact, the static state model fails to fit the distribution histograms of larger t.w. because of more frequent transitions within dynamic systems. A first attempt to fit the experimental S G /S R distribution histograms of the same data set for t.w.=2, 3 and 4 ms, with the model of three static populations of different FRET efficiencies (or distances) did not provide a satisfying result. Consequently, we conclude that the molecules are dynamic on a timescale below 4 ms. Then, a model that accounts for two static species (high FRET (Resting) state, S G /S R =0.2 and low FRET (Active) state S G /S R =3), and dynamic species interconverting between these states ( S G /S R =0.8–1.2, depending on the ligand) was applied, and allowed for an accurate description of the experimental S G /S R distribution. In order to determine the reproducibility of the data, measurements were performed ten times. The FRET-derived mean distances and the standard deviations for the Resting and Active states are 28.4±0.8 and 56.1±0.8 Å, respectively. By applying rigorous experimental calibration procedures, the average distances and errors obtained from different high precision-FRET measurements have only minimal variations, and hence, a high degree of statistical confidence in the discrimination between the states. It should be pointed out that even if the considered model overall relatively well describes the data histograms, the slower than 4 ms exchange within the populations of resting (R) and an active (A) states are possible, which we cannot identify in our experiments. Correlation analysis 2cFCCS and fFCS analysis are extensively described in Supplementary Note . Statistical analysis Statistical analyses were performed on at least six to ten individual data sets and the means±s.e.m are shown as histograms. * P -value<0.05, ** P -value<0.01 and *** P -value<0.001, NS, non-significant. How to cite this article: Olofsson, L. et al. Fine tuning of sub-millisecond conformational dynamics controls metabotropic glutamate receptors agonist efficacy. Nat. Commun. 5:5206 doi: 10.1038/ncomms6206 (2014).